Modular total syntheses oftrans-clerodanes and sesquiterpene (hydro)quinones via tail-to-head cyclization and reductive coupling strategies 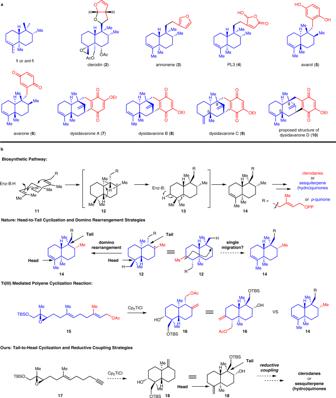Fig. 1: Selectedtrans-clerodanes and sesquiterpene (hydo)quinones, the hypothesis of the biogenesis of such structures and our synthetic strategies. aSelectedtrans-clerodanes and sesquiterpene (hydo)quinones that feature the similartrans-decalin core structure1orent-1.bNature’s head-to-tail cyclization and domino rearrangement strategies to synthesizetrans-clerodanes and some sesquiterpene (hydo)quinones. Our’s tail-to-head cyclization and reductive coupling strategies to synthesize these types of natural products. The trans -clerodanes and sesquiterpene (hydro)quinones are a growing class of natural products that exhibit a wide range of biological activities. Although they are different types of natural products, some of them feature the same trans -decalin core structure. Here, we report the total syntheses of two members of trans -clerodanes, five members of sesquiterpene (hydro)quinones as well as the proposed structure of dysidavarone D via a modular synthetic route. A bioinspired tail-to-head cyclization strategy was developed to syntheses of the trans -decalin architectures by using two diastereochemically complementary radical polyene cyclization reactions catalyzed by Ti(III) and mediated by Mn(III), respectively. The different types of side chains were introduced by challenging nickel catalyzed reductive couplings of sterically hindered alkyl halides. The synthesis of the proposed dysidavarone D proved a wrong structural assignment of the natural product. The trans -clerodanes and sesquiterpene (hydro)quinones are different types of natural products, both of which exhibit a wide range of biological activities [1] , [2] , [3] . However, some of them ( 2 – 10 , Fig. 1a ) feature the same trans -decalin core structure ( 1 or ent - 1 , Fig. 1a ) [4] , [5] , [6] , [7] , [8] , [9] , [10] , [11] , [12] , [13] , [14] , [15] , [16] , [17] , [18] , [19] , [20] , [21] , [22] , [23] , [24] , [25] , [26] . It suggests that these might have a similar biosynthetic pathway in Nature. As shown in Fig. 1b , the trans -decalin skeleton was proposed to generate by cyclases catalyzed proton-initiated cationic polyene cyclization followed by a series of Wagner-Meerwein rearrangements [1] , [2] . The biosynthetic pathway could be divided into two stages–the head-to-tail cyclization stage ( 11 – 12 ) and the domino rearrangement stage ( 12 – 14 ). The trans -decalin structure (highlighted in blue) of the cyclization intermediate 12 , if redrawn in alternative orientation, is similar to the domino rearrangement product 14 . The only difference is the position of the methyl groups (highlighted in red). We envisioned whether 12 could be transformed into 14 by a “single migration”. Titanium(III) mediated radical cyclization of epoxy alkenes was originally developed by RajanBabu and Nugent [27] which was then expanded to radical polyene cyclization and extensively used in the total synthesis of natural products [28] . Comparison of the structure of 14 and 16 —the titanium(III) mediated radical polyene cyclization product of the derivative of farnesol 15 [29] , [30] , [31] , [32] , both of them also have similar trans -decalin architecture (in blue). If the acetate and the methylene (in red) in 16 , which were generated from the acetate and methyl group (the red part) in 15 , were removed and the hydroxyl group was transformed into a methyl group, the trans -decalin architecture of trans -clerodanes and sesquiterpene (hydro)quinones could be delivered. We think that if the acetate and methyl group in 15 are pre-removed, the desired cyclization product may be obtained without the redundant acetate and methylene group. With this thought in mind, we designed the cyclization precursor 17 . After titanium(III)-mediated radical polyene cyclization and introduction of the desired methyl group from the secondary hydroxyl group, the previously mentioned “single migration” to construct the trans -decalin core structure of trans -clerodanes and sesquiterpene (hydro)quinones could be achieved—this is a key differentiation from biosynthetic pathway where the cyclization of 17 initiated from the tail of the natural products and ended at the head. At last, the different types of side chains could be installed by nickel-catalyzed sterically hindered reductive couplings [33] , [34] , [35] that enables the modular route to this type of natural product. Herein, we report the total syntheses of 3 – 10 based on the tail-to-head cyclization and the reductive coupling strategies. Fig. 1: Selected trans -clerodanes and sesquiterpene (hydo)quinones, the hypothesis of the biogenesis of such structures and our synthetic strategies. a Selected trans -clerodanes and sesquiterpene (hydo)quinones that feature the similar trans -decalin core structure 1 or ent - 1 . b Nature’s head-to-tail cyclization and domino rearrangement strategies to synthesize trans -clerodanes and some sesquiterpene (hydo)quinones. Our’s tail-to-head cyclization and reductive coupling strategies to synthesize these types of natural products. Full size image The syntheses of annonene and PL-3 We first investigated our strategies in the total synthesis of trans -clerodanes (Fig. 2 ). Starting from the allylic alcohol 19 (one step from geranyl acetate), Sharpless epoxidation with (−)-diethyl D -tartrate (( D )-DET), Ti(O i -Pr) 4 and t -butyl hydroperoxide (TBHP) introduced the initial chiral center followed by one pot protection of the alcohol with t -butyldimethylsilyl chloride (TBSCl) afforded the epoxide 20 in 93% yield. 20 was subjected to a copper (Li 2 CuCl 4 ) catalyzed coupling reaction with Grignard reagent 21 to assemble the alkyne chain, and subsequent one-pot deprotection of the trimethylsilyl (TMS) with K 2 CO 3 and methanol (MeOH) to deliver cyclization precursor 17 in 72% yield [36] . With 17 in hand, the titanium(III) catalyzed radical polyene cyclization was investigated. Previous research indicated that this type of radical polyene cyclization could be achieved by using two equivalents of Cp 2 TiCl at 60 °C, yet no catalytic reaction was reported [37] . Inspired by Gansäuer’s work [38] , and Nugent and RajanBabu’s recent essay [39] , we found that the radical polyene cyclization could proceed smoothly to generate 18 in 65% yield when treatment of 17 with 0.2 equiv of Cp 2 TiCl 2 , 2.5 equiv of 2,4,6-collidine·HCl and 3.0 equiv of Zn at 40 °C. The 2,4,6-collidine·HCl played important roles in the catalytic reaction. Not only as the proton source to regenerate the Cp 2 TiCl 2 from the intermediate, but 2,4,6-collidine·HCl could also interact with Cp 2 TiCl to form a complex which could decrease the transient concentration of free Cp 2 TiCl [39] , [40] , [41] . This effect could arrest the disproportionation of the initial radical whose rate is dependent on the concentration of Cp 2 TiCl. Pressing forward, exposure of 18 to Ley’s oxidation conditions enabled the oxidation of secondary alcohol to a ketone. Subsequent Wittig reaction of the resultant ketone followed by one-pot deprotection of the t -butyldimethylsilyl (TBS) with tetrabutylammonium fluoride (TBAF) gave alcohol 22 in 49% yield over 2 steps. Next, in anticipation of probing the projected reductive coupling, alcohol 22 was transformed into bromide 23 in 39% overall yield through hydroxyl group directed hydrogenation of one of the terminal alkenes with Crabtree’s catalyst [42] , [43] and one-pot isomerization of another terminal alkene with Co(Sal t -Bu , t -Bu )Cl and PhSiH 3 [44] , followed by bromination of the hydroxyl group with CBr 4 and Ph 3 P. Pleasingly, we found that the desired reductive coupling of 23 with 24 to generate annonene ( 3 ) could indeed be effected using Shu’s conditions [NiBr 2 , Mn, (4-CF 3 Ph) 3 P] [45] . Photosensitized oxidation of 3 [O 2 , Rose Bengal, N , N -diisopropylethylamine (DIPEA), visible light] gave 16-hydroxycleroda-3,13-dien-15,16-olide (PL-3, 4 ) in 78% yield through the [4 + 2] addition of singlet oxygen to the 3-alkylfuran and regiospecific deprotonation [46] , [47] . Fig. 2: Syntheses of annonene and PL3. Reagents and conditions: a ( D )-DET (0.1 equiv), Ti(O i -Pr) 4 (0.05 equiv), TBHP (1.5 equiv, 5.5 M in decane), 3 Å MS, CH 2 Cl 2 , −30 °C, 12 h, then TBSCl (2.0 equiv), imidazole (3.0 equiv), 0 °C, 1 h, 93%; b 21 (1.5 equiv), Li 2 CuCl 4 (0.1 equiv), THF, 0 °C, 1 h, then K 2 CO 3 (10.0 equiv), MeOH:THF = 1.5:1, 23 °C, 12 h, 72%; c Cp 2 TiCl 2 (0.2 equiv), Zn (3.0 equiv), 2,4,6-collidine·HCl (2.5 equiv), THF, 40 °C, 3 h, 65%; d TPAP (0.1 equiv), NMO (2.0 equiv), 4 Å MS, CH 2 Cl 2 , 23 °C, 1 h, 82%; e NaHMDS (1.5 eqiv), Ph 3 PCH 3 Br (1.75 equiv), THF, 60 °C, 8 h, then TBAF (5.0 equiv), 4 h, 60%; f [Ir(cod)(Py)(PCy 3 )] + PF 6 − (0.005 equiv), H 2 , CH 2 Cl 2 , 23 °C, 2 h, then Co(Sal t -Bu, t -Bu )Cl (0.05 equiv), PhSiH 3 (0.2 equiv), benzene, 23 °C, 8 h, 73%; g CBr 4 (2.0 equiv), PPh 3 (3.0 equiv), Py, 60 °C, 4 h, 53%; h 24 (3.0 equiv), NiBr 2 (0.3 equiv), Mn (4.0 equiv), P(4-CF 3 Ph) 3 (0.3 equiv), DMF:DMSO = 1:1, 60 °C, 16 h, 50%; i Rose·Bengal (0.025 equiv), DIPEA (10.0 equiv), tungsten lamp (200 W), CH 2 Cl 2 , −78 °C, 3 h, 78%. ( D )-DET (−)-diethyl D -tartrate, TBHP t -butyl hydroperoxide, MS molecular seives, TBSCl t -butyldimethylsilyl chloride, THF tetrahydrofuran, TPAP tetrapropylammonium perruthenate, NMO 4-methylmorpholine N -oxide, NaHMDS sodium bis(trimethylsilyl)amide, DMF N,N -dimethylformamide; DMSO dimethyl sulfoxide, TBAF tetrabutylammonium fluoride, DIPEA N -ethyldiisopropylamine. Full size image The syntheses of avarone and avarol Having successfully completed the total syntheses of annonene and PL-3, we applied the above strategies to the syntheses of avarone and avarol (Fig. 3 ). Compound 25 was synthesized from geranyl acetate in a similar fashion to that described above in 7 steps in 11% overall yield. Iodination of the hydroxyl group with Ph 3 P and I 2 afforded iodide 26 in 61% yield. NiI 2 catalyzed reductive coupling of 26 and 3-bromo-phenol ( 27 ) gave 29 in 63% yield [48] , [49] , [50] , [51] . Lastly, oxidation of the resultant phenol with salcomine and O 2 provided avarone ( 6 ) in 71% yield [52] , [53] , while quenching with an aqueous solution of Na 2 S 2 O 4 led to avarol ( 5 ) in 63% yield. Fig. 3: Syntheses of avarone and avarol. Reagents and conditions: a I 2 (2.0 equiv), Imidazole (3.0 equiv), PPh 3 (3.0 equiv), benzene, 50 °C, 12 h, 61%; b 27 (3.0 equiv), NiI 2 (0.2 equiv), 28 (0.2 equiv), Zn (3.0 equiv), DMAc, 80 °C, 2 h, 63%; c salcomine (2.5 equiv), O 2 , DMF, 40 °C, 2 days, 71%; d salcomine (2.5 equiv), O 2 , DMF, 40 °C, 2 days, then aqueous Na 2 S 2 O 4 , 63%. DMAc dimethylacetamide. Full size image The syntheses of dysidavarones A, B and C The strategies were then applied to the syntheses of dysidavarones A, B and C ( 7 – 9 ) which possess tetracyclic frameworks (Fig. 4 ). Compound 30 could also be synthesized from geranyl acetate in a similar fashion to that described above in 5 steps in 25% overall yield. 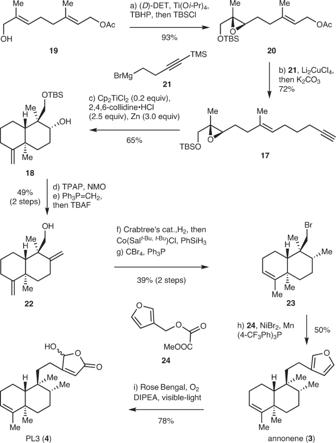Fig. 2: Syntheses of annonene and PL3. Reagents and conditions:a(D)-DET (0.1 equiv), Ti(Oi-Pr)4(0.05 equiv), TBHP (1.5 equiv, 5.5 M in decane), 3 Å MS, CH2Cl2, −30 °C, 12 h, then TBSCl (2.0 equiv), imidazole (3.0 equiv), 0 °C, 1 h, 93%;b21(1.5 equiv), Li2CuCl4(0.1 equiv), THF, 0 °C, 1 h, then K2CO3(10.0 equiv), MeOH:THF = 1.5:1, 23 °C, 12 h, 72%;cCp2TiCl2(0.2 equiv), Zn (3.0 equiv), 2,4,6-collidine·HCl (2.5 equiv), THF, 40 °C, 3 h, 65%;dTPAP (0.1 equiv), NMO (2.0 equiv), 4 Å MS, CH2Cl2, 23 °C, 1 h, 82%;eNaHMDS (1.5 eqiv), Ph3PCH3Br (1.75 equiv), THF, 60 °C, 8 h, then TBAF (5.0 equiv), 4 h, 60%;f[Ir(cod)(Py)(PCy3)]+PF6−(0.005 equiv), H2, CH2Cl2, 23 °C, 2 h, then Co(Salt-Bu,t-Bu)Cl (0.05 equiv), PhSiH3(0.2 equiv), benzene, 23 °C, 8 h, 73%;gCBr4(2.0 equiv), PPh3(3.0 equiv), Py, 60 °C, 4 h, 53%;h24(3.0 equiv), NiBr2(0.3 equiv), Mn (4.0 equiv), P(4-CF3Ph)3(0.3 equiv), DMF:DMSO = 1:1, 60 °C, 16 h, 50%;iRose·Bengal (0.025 equiv), DIPEA (10.0 equiv), tungsten lamp (200 W), CH2Cl2, −78 °C, 3 h, 78%. (D)-DET (−)-diethylD-tartrate, TBHPt-butyl hydroperoxide, MS molecular seives, TBSClt-butyldimethylsilyl chloride, THF tetrahydrofuran, TPAP tetrapropylammonium perruthenate, NMO 4-methylmorpholineN-oxide, NaHMDS sodium bis(trimethylsilyl)amide, DMFN,N-dimethylformamide; DMSO dimethyl sulfoxide, TBAF tetrabutylammonium fluoride, DIPEAN-ethyldiisopropylamine. Deprotection of TBS ether with HF·py followed by iodination of the resultant hydroxyl group afforded the iodide 31 in 65% yield over two steps. The reductive coupling of 31 and 32 was achieved under the NiBr 2 ·DME catalyzed conditions [48] , [49] , [50] , [51] . Subsequent palladium [NHC-Pd(II)-Im] catalyzed intramolecular α -arylation of ketone to assemble the bicyclo[3.3.1] architecture provided 33 in 38% overall yield [54] . The stereochemistry of 33 was unambiguously confirmed by the X-ray crystallographic analysis. Compound 33 was then converted into quinone 34 in 64% overall yield through Wittig reaction and removal of methyl protection group by n -BuSLi [55] , followed by the oxidation of the resultant phenol to quinone with salcomine and O 2 [52] , [53] . The ethoxy group in dysidavarones was introduced by treating 34 with Et 3 N in ethanol (EtOH) under O 2 [56] , [57] , affording dysidavarone C ( 9 ) and 35 in 19% and 25% yield, respectively. Isomerization of terminal alkene in 9 under acidic conditions [ p -toluenesulfonic acid monohydrate (PTSA·H 2 O), acetic acid (HOAc)] provided dysidavarone B ( 8 ) in 54% yield [25] . Dysidavarone A ( 7 ) could also be obtained from 35 under the same conditions in 63% yield. Fig. 4: Syntheses of dysidavarones A–C. Reagents and conditions: a HF·Py:THF = 1:4, 40 °C, 2 h, 73%; b I 2 (2.0 equiv), PPh 3 (3.0 equiv), benzene, 23 °C, 16 h, 89%; c 32 (3.0 equiv), 28 (0.2 equiv), NiBr 2• DME (0.2 equiv), Mn (3.0 equiv), DMAc, 23 °C, 16 h; d NHC-Pd(II)-Im (0.2 equiv), t -BuONa (3.0 equiv), 1,4-dioxane, 110 °C, 3 h, 38% (2 steps); e CH 3 PPh 3 Br (10.0 equiv), t -BuOK (10.0 equiv), toluene, 120 °C, 7 h, 88%; f n -BuSH (10.0 equiv), n -BuLi (10.0 equiv), HMPA, 110 °C, 4 h, 85%; g salcomine (3.0 equiv), O 2 , acetonitrile, 23 °C, 85%; h Et 3 N (50.0 equiv), O 2 , EtOH, 30 °C, 9 , 19%, 35 , 25%; i PTSA·H 2 O (0.2 equiv), HOAc, 40 °C, 8 , 54%, 7 , 63%. 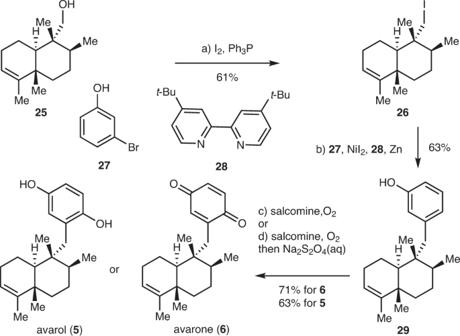Fig. 3: Syntheses of avarone and avarol. Reagents and conditions:aI2(2.0 equiv), Imidazole (3.0 equiv), PPh3(3.0 equiv), benzene, 50 °C, 12 h, 61%;b27(3.0 equiv), NiI2(0.2 equiv),28(0.2 equiv), Zn (3.0 equiv), DMAc, 80 °C, 2 h, 63%;csalcomine (2.5 equiv), O2, DMF, 40 °C, 2 days, 71%;dsalcomine (2.5 equiv), O2, DMF, 40 °C, 2 days, then aqueous Na2S2O4, 63%. DMAc dimethylacetamide. DME 1,2-dimethoxyethane, HMPA hexamethylphosphoramide, PTSA·H 2 O p -toluenesulfonic acid monohydrate. Full size image The synthesis of proposed structure of dysidavarone D Dysidavarone D also features a tetracyclic framework similar to dysidavarones A–C, however, the stereochemistry is different which methyl groups at C5 and C9 position of the trans -decalin architecture are trans -form. Unfortunately, efforts to construct the trans -decalin architecture of dysidavarone D via titanium(III) catalyzed radical polyene cyclization were unfruitful [58] . As a result, we developed an alternate tail-to-head cyclization route to synthesize dysidavarone D by a Mn(OAc) 3 ·2H 2 O mediated radical polyene cyclization (Fig. 5 ) [59] . Allylation of the bisenolate of 37 with allyl bromide 36 delivered 38 (73% yield), which was subjected to the Mn(OAc) 3 ·2H 2 O mediated radical polyene cyclization conditions to give keto ester 39 (61% yield). The keto ester 39 was then converted into iodide 40 through the protection of the ketone by transforming it into enol methyl ether, LiAlH 4 reduction of the ester to primary alcohol followed by one-pot hydrolysis of methyl enol ether to ketone, and iodination of the resultant hydroxyl group. Due to the cis configuration of the C5-methyl group and the C9-iodomethyl group, the reductive coupling of iodide 40 and 32 would be more challenging than previous substrates. Catalytic conditions only afforded a trace amount of coupling product. After extensive optimization, we found that 1.5 equiv of NiBr 2 ·DME and ligand 28 could promote the desired reductive coupling with acceptable efficiency. Subsequent isomerization of the terminal alkene delivered 41 in 21% overall yield. Quinone 42 was synthesized from 41 in a similar fashion to that described above in the syntheses of dysidavarones A–C in 4 steps. The stereochemistry of the tetracyclic framework was unambiguously confirmed by the X-ray crystallographic analysis of the intramolecular α -arylation product of ketone 41 (see Supplementary Information ). The introduction of the ethoxy group was achieved by treating 42 with Co(OAc) 2 in EtOH under O 2 , delivering a 1:1 mixture of inseparable regioisomers in 42% yield (70% yield based on recovered starting material) [60] . The resulting quinone mixtures were reduced to hydroquinones, followed by selective mono-TBS-protection generated silyl ethers 43 and 44 in 37% and 26% yield, respectively, which were separable at this stage. The position of ethoxy groups in 43 and 44 was unambiguously confirmed by its nuclear Overhauser effect spectroscopy (NOESY) spectra. 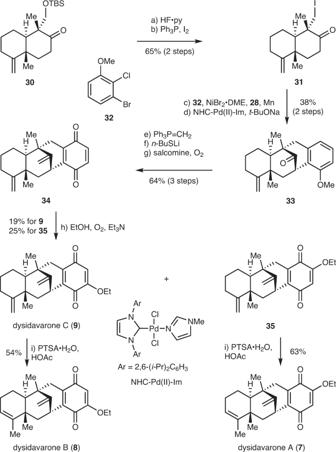Fig. 4: Syntheses of dysidavarones A–C. Reagents and conditions:aHF·Py:THF = 1:4, 40 °C, 2 h, 73%;bI2(2.0 equiv), PPh3(3.0 equiv), benzene, 23 °C, 16 h, 89%;c32(3.0 equiv),28(0.2 equiv), NiBr2•DME (0.2 equiv), Mn (3.0 equiv), DMAc, 23 °C, 16 h;dNHC-Pd(II)-Im (0.2 equiv),t-BuONa (3.0 equiv), 1,4-dioxane, 110 °C, 3 h, 38% (2 steps);eCH3PPh3Br (10.0 equiv),t-BuOK (10.0 equiv), toluene, 120 °C, 7 h, 88%;fn-BuSH (10.0 equiv),n-BuLi (10.0 equiv), HMPA, 110 °C, 4 h, 85%;gsalcomine (3.0 equiv), O2, acetonitrile, 23 °C, 85%;hEt3N (50.0 equiv), O2, EtOH, 30 °C,9, 19%,35, 25%;iPTSA·H2O (0.2 equiv), HOAc, 40 °C,8, 54%,7, 63%. DME 1,2-dimethoxyethane, HMPA hexamethylphosphoramide, PTSA·H2Op-toluenesulfonic acid monohydrate. 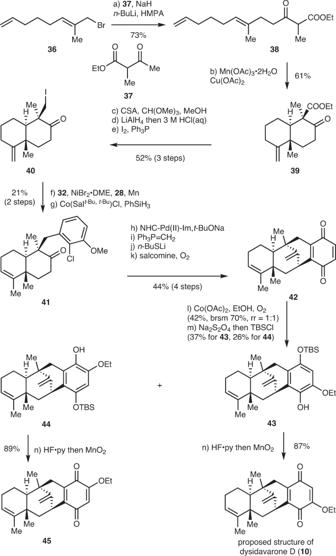Fig. 5: Synthesis of proposed structure of dysidavarone D. Reagents and conditions:aNaH (5.0 equiv),n-BuLi (5.0 equiv),37(5.0 equiv), HMPA (1.2 equiv), THF, 23 °C, 1 h, 73%;bMn(OAc)3·2H2O (2.0 equiv), Cu(OAc)2(1.1 equiv), AcOH, 40 °C, 24 h, 61%;cCH(OMe)3(7.5 equiv), CSA (0.10 equiv), MeOH, 23 °C, 4.5 h, 81%;dLiAlH4(4.0 equiv), THF, 15 h, then 3 M HCl, 23 °C, 1 h, 75%;ePPh3(1.3 equiv), I2(1.2 equiv), imidazole (2.0 equiv), benzene, 40 °C, 15 h, 85%;fNiBr·DME (1.5 equiv),28(1.5 equiv), Mn (3.0 equiv),32(3.0 equiv), DMAc, 17 h;gCo(Salt-Bu,t-Bu)Cl (0.05 equiv), PhSiH3(0.2 equiv), benzene, 23 °C, 24 h, 21% (2 steps);hNHC-Pd(II)-Im (0.1 equiv),t-BuONa (3.0 equiv), 1,4-dioxane, 110 °C, 6 h, 65%;it-BuOK (10.0 equiv) PPh3CH3Br (10.0 equiv), toluene, 120 °C, 8 h, 91%;jn-BuSH (7.5 equiv),n-BuLi (7.5 equiv), HMPA, 110 °C, 89%;ksalcomine (3.0 equiv), O2, acetonitrile, 23 °C, 3 h, 83%;lCo(OAc)2(3.0 equiv), O2,EtOH, 160 °C, 10 h, 42% (b.r.m. 70%, r.r. = 1:1);maqueous Na2S2O4, THF, 1 h, then imidazole (5.0 equiv), TBSCl (3.0 equiv), DCM, −10 °C, 37% for43, 26% for44; andnHF·Py:THF = 1:2, 23 °C, 1 h, then MnO2, CH2Cl2, 23 °C, 15 min, 87% for proposed structure of dysidavarone D (10), 89% for45. Lastly, 43 and 44 were converted into corresponding quinones 10 and 45 in 87% and 89% yield, respectively, through deprotection of TBS with HF·py following oxidation of the resultant hydroquinones to quinones with MnO 2 [61] . However, neither NMR spectra of 10 nor 45 matched with the originally proposed structure of dysidavarone D, suggesting the original structural assignment may be incorrect [15] . Fig. 5: Synthesis of proposed structure of dysidavarone D. Reagents and conditions: a NaH (5.0 equiv), n -BuLi (5.0 equiv), 37 (5.0 equiv), HMPA (1.2 equiv), THF, 23 °C, 1 h, 73%; b Mn(OAc) 3 ·2H 2 O (2.0 equiv), Cu(OAc) 2 (1.1 equiv), AcOH, 40 °C, 24 h, 61%; c CH(OMe) 3 (7.5 equiv), CSA (0.10 equiv), MeOH, 23 °C, 4.5 h, 81%; d LiAlH 4 (4.0 equiv), THF, 15 h, then 3 M HCl, 23 °C, 1 h, 75%; e PPh 3 (1.3 equiv), I 2 (1.2 equiv), imidazole (2.0 equiv), benzene, 40 °C, 15 h, 85%; f NiBr·DME (1.5 equiv), 28 (1.5 equiv), Mn (3.0 equiv), 32 (3.0 equiv), DMAc, 17 h; g Co(Sal t -Bu, t -Bu )Cl (0.05 equiv), PhSiH 3 (0.2 equiv), benzene, 23 °C, 24 h, 21% (2 steps); h NHC-Pd(II)-Im (0.1 equiv), t -BuONa (3.0 equiv), 1,4-dioxane, 110 °C, 6 h, 65%; i t -BuOK (10.0 equiv) PPh 3 CH 3 Br (10.0 equiv), toluene, 120 °C, 8 h, 91%; j n -BuSH (7.5 equiv), n -BuLi (7.5 equiv), HMPA, 110 °C, 89%; k salcomine (3.0 equiv), O 2 , acetonitrile, 23 °C, 3 h, 83%; l Co(OAc) 2 (3.0 equiv), O 2, EtOH, 160 °C, 10 h, 42% (b.r.m. 70%, r.r. = 1:1); m aqueous Na 2 S 2 O 4 , THF, 1 h, then imidazole (5.0 equiv), TBSCl (3.0 equiv), DCM, −10 °C, 37% for 43 , 26% for 44 ; and n HF·Py:THF = 1:2, 23 °C, 1 h, then MnO 2 , CH 2 Cl 2 , 23 °C, 15 min, 87% for proposed structure of dysidavarone D ( 10 ), 89% for 45 . Full size image In conclusion, we have accomplished the total syntheses of a number of trans -clerodanes and sesquiterpene (hydro)quinones through tail-to-head cyclization and reductive coupling strategies. The synthesis of the proposed dysidavarone D also suggested incorrect structural assignments from the previous report. We believe that the flexible, modular, and generalized biomimetic [62] synthetic route may facilitate biological studies of these natural products and their derivatives. All reactions were carried out under an argon atmosphere with dry solvents under anhydrous conditions unless otherwise noted. Tetrahydrofuran (THF), diethyl ether (Et 2 O), and toluene were distilled immediately before use from sodium-benzophenone ketyl. Dimethylformamide (DMF) and dichloromethane (CH 2 Cl 2 ) were distilled from calcium hydride and stored under an argon atmosphere. Yields refer to chromatographically and spectroscopically ( 1 H and 13 C NMR) homogeneous materials unless otherwise stated. Reagents were purchased at the highest commercial quality and used without further purification unless otherwise stated. Reactions were magnetically stirred and monitored by thin-layer chromatography (TLC) carried out on 0.25 mm Xinnuo silica gel plates (60F-254) using UV light as a visualizing agent, and an ethanolic solution of phosphomolybdic acid and cerium sulfate, and heat as developing agents. Steema silica gel (60, academic grade, particle size 0.040–0.063 mm) was used for flash column chromatography. Preparative thin-layer chromatography separations were carried out on 0.50 mm Xinuo silica gel plates (60F-254). NMR spectra were recorded on Bruker 600 MHz and 400 MHz instruments and calibrated using residual undeuterated solvent as an internal reference. The following abbreviations were used to explain the multiplicities: s = singlet, d = doublet, t = triplet, q = quartet, m = multiplet. IR spectra were recorded on a Perkin-Elmer 1000 series FT-IR spectrometer. High-resolution mass spectra (HRMS) were recorded on an Agilent 6244 Tof-MS using ESI (Electrospray Ionization).